Coupling unstable agents in biological control It has long been a goal of farm policy to manage production in such a way that expensive off-farm inputs and negative environmental consequences can be simultaneously minimized. One generalized philosophy that has gained currency in recent years is autonomous pest control, in which complex ecological interactions are encouraged to maintain the ecosystem in a state of permanence with the pest below economic thresholds. Early experience with biological control was hampered significantly by the inherent instability of many of the control agents, suggesting that pursuit of the autonomous strategy could be difficult. Here we show that combining two unstable two-dimensional systems (pest–predator and pest–pathogen) produces a stable three-dimensional system (pest–predator–pathogen) that is robust to perturbations in initial conditions. Contrary to expectations, the inclusion of negative interactions, which are arguably a necessary consequence of increased complexity, can stabilize unstable conditions and rescue biological control of simpler, ineffective pest management systems. Charles Elton [1] first juxtaposed the striking stability of natural systems and the plagues of diseases and pests so common in agricultural systems in 1958. Since then, there have been many attempts to mimic such natural systems in agriculture by releasing natural enemies of pests as biological control agents to capture the control mechanisms that presumptively led to the stability of natural systems [2] . However, both in practice and theory, biological control was difficult to stabilize [3] , [4] , [5] , [6] . Generalist control agents often had non-target negative effects on other beneficial insects, whereas specialist control agents disappeared as their target pest resource was eliminated [7] , [8] . This often led to secondary resurgence of the pest once the agent was gone, followed by an inundation of the system with more agents as they disappeared—a very costly solution [9] . These practical issues mirrored debates in the theoretical literature. In the paradox of biological control, simple predator–prey theory was used to show that the most efficient control agents caused the most extreme pest outbreaks, since efficient agents overexploited resources and died quickly, allowing pests to resurge in great numbers while agent populations slowly recovered [5] . In another example, the Nicholson–Bailey model sparked controversy since its original form, which used difference equations to describe parasitoid–host interactions, was incapable of stable interactions, and only through extensive revisions incorporating complexities of host–parasite biology was it forced to do so [4] . One overarching theme that resulted from this work was that strong interactions tend to destabilize pest control. We define unstable to mean any pest population that becomes too extreme or variable to be practical for a farmer. This is an assigned threshold beyond which damage caused by pests to crops become economically unsustainable [5] , [10] . Control agents are often designed to strongly inhibit pest growth, yet these kinds of strong consumer–resource interactions are often themselves, unstable [5] , [11] . Most recently, theoretical work utilizing food web modules have found that weak predator–prey interactions can help stabilize unstable systems [12] . These models show that unpredictable, chaotic dynamics can be dampened into stable equilibria by the imposition of a stable consumer–resource interaction [12] . However, since agricultural pests are defined by their propensity for unstable growth, and pests remain a major agricultural problem, it stands to reason that unstable interactions between pests and natural enemies are more common [13] . However, the question of whether two unstable interactions can be combined to produce stability has yet to be asked. If possible, then a diverse assemblage of separately unstable control agents could be combined to create a functional pest management programme, reminiscent of the stability that Elton first noticed in natural systems [1] . In addition, there has always been a disjunction between the theory of competitive exclusion and the coexistence of multiple competing natural enemies in nature that has been explained, in recent literature, through mechanisms of species complementarity, where enemies split a shared resource into separate niches, thus preventing direct competition [14] . Although there exists strong evidence that complementarity between diverse assemblages of organisms (mostly grasses and so on) may lead to stability of ecosystems in the biodiversity–ecosystem function literature, empirical evidence for complementarity in biological control is not abundant [15] , [16] , [17] . Many positive effects of natural enemy diversity on biological control are reported, but evidence tends to favour sampling effects from one strong control agent, or insurance effects where many redundant enemies buffer systems from rapid changes in the environment [16] , [17] , [18] , [19] , [20] , [21] . In contrast, competition over shared resources and predation among natural enemies (intraguild predation (IGP)) are very common but almost automatically suspected of impairing biological control in empirical work and coexistence in theoretical models [16] , [17] , [22] , [23] , [24] , [25] , [26] . However, proponents of autonomous biological control argue that these same negative interactions are a natural consequence of a complex network of multiple natural enemies, and may actually help suppress pest problems by acting as a system of checks and balances limiting overexploitation by any one enemy—essentially reconciling the disjunction [27] , [28] . To the extent studied thus far, all herbivores are attacked by both predators/parasitoids and pathogens [26] , [29] , [30] , [31] , [32] , suggesting that any system of autonomous control will automatically contain this duality of control factors. Thus, we investigate the controlling effects of first a pathogen, then a predator and finally their combination. Recently, scientists have encouraged the utilization of predators and pathogens in biological control, arguing that facilitation is more likely than competition because of differences in size, life cycles and modes of attack [29] . However, in cases where pathogens and predators are not separated by space or time, we argue that the potential for strong negative interactions is high, especially considering the evidence of non-target effects by generalist pathogens on other competing natural enemies, primarily predators [26] , [31] . Although studies more frequently report cases of IGP between predators, the prevalence of coexisting disease and predator control agents suggests that predators must engage in IGP with pathogens whenever they happen to consume infected prey [17] , [30] , [31] , [32] . We argue that in cases where infection of hosts is widespread or latent for long periods of time [33] , prey choice becomes limited for predators, making IGP more likely [30] . One well-documented example is the predation of pests that harbour developing parasitoids [32] . The same argument can be made for developing fungal spores within pests, although few have attempted to test this question [30] , [31] . Currently, IGP is generally considered a hindrance to biocontrol efforts, and is often used as a default explanation for non-significant or negative relationships between diversity of control agents and biocontrol [16] , [18] , [19] , [20] , [22] , [23] , while in the theoretical literature IGP is presented as a hindrance to competitive coexistence by seeming on the surface to lead to exclusion of the intraguild prey [17] , [24] , [25] , [26] . In consideration of the strong negative interactions that may occur among control agents used in tandem for biological control, we combine standard Rosenzweig/MacArthur [34] and epidemic models [35] following examples in the mathematical biology literature [36] , [37] , [38] , [39] , [40] , [41] , [42] and modify them to determine whether combining two ineffective control agents (ineffective in the sense that pests remain permanently in an outbreak mode) through strong competition over a shared resource and IGP can rescue control. We find that stability can indeed be rescued, forcing us to reassess current generalizations on the effects of strong negative interspecific interactions on ecosystem stability. Model justification In agricultural systems where crops are carefully managed, resources are rarely limiting for pests since most pest-control strategies are enacted before crop yields drop to the point where pests experience density dependence [10] . We therefore retain density independence on the prey, since we are concerned with the alternate control by disease or predator, not with some form of bottom up or otherwise control (which would be implied by including the customary ‘carrying capacity’ of the prey). However, in acknowledgement of the fact that competitive exclusion between the control agents is inevitable without some form of nonlinearity [43] , [44] , [45] , we instill density dependence on the predator following the example of a previous predator–prey model [46] . We choose to impose density dependence on the predator rather than the pathogen by reasoning that non-food resources such as space or nesting habitat are more likely limited in predators than pathogens due to size alone (Methods). Thus we begin with a model where both the disease (Methods, equations (1a) and (1b)) and predator (Methods, equations (2a) and (2b)) acting alone are able to control the pest, but where the pest can, under certain circumstances, escape control from either agent ( Fig. 1b,d ). We take control and stability to mean any pest population that ultimately coalesces to some constant or oscillating size consistently below pest tolerance thresholds ( Fig. 1a,c ) [10] . For our purposes, we set tolerance thresholds to a value of 500 susceptible pest individuals after 10,000 generations. Although the specific threshold is arbitrary, the long timescale allows us to see whether populations ultimately tend towards ∞, −∞ (unstable) or consistently remain within biologically realistic values (stable). 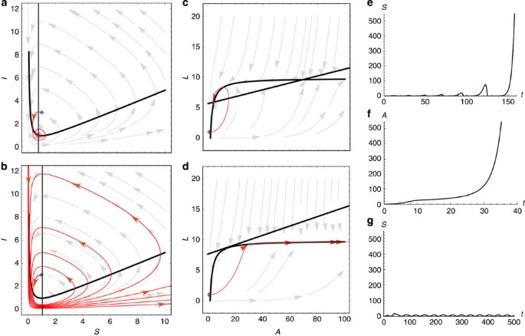Figure 1: Taking unstable conditions to stable ones. Pest individuals (SorA) plotted against enemy individuals (I-pathogen orL-predator) yield phase portraits of example (a) stable and (b) unstable dynamics for subsystem 1: pathogen–pest and (c) stable and (d) unstable dynamics for subsystem 2: predator–pest. Dark black lines are zero growth isoclines, grey arrows indicate the vector field and red arrows are exemplary trajectories from initial conditions indicated by a grey dot. Corresponding time series plots for unstable subsystems 1 (e) and 2 (f), and the result of combiningeandfto produce (g) system 3 (pathogen–predator–pest). The parameter values are:r=0.46,α1=0.9,α2=0.06,β1=1,β2=0.01,m1=0.47,m2=0.1,K=10 andε=0.8, and the initial conditions areS0=1,I0=3 andL0=1ris the per capita growth rate of the pest,α1andα2are the attack rates of the pathogen and the predator, respectively,β1andβ2are the handling times of the pathogen and predator, respectively,m1andm2are the mortality rates of the pathogen and predator, respectively,Kis the carrying capacity of the predator andεis the conversion rate of infected prey consumed to predators produced. Figure 1: Taking unstable conditions to stable ones. Pest individuals ( S or A ) plotted against enemy individuals ( I -pathogen or L -predator) yield phase portraits of example ( a ) stable and ( b ) unstable dynamics for subsystem 1: pathogen–pest and ( c ) stable and ( d ) unstable dynamics for subsystem 2: predator–pest. Dark black lines are zero growth isoclines, grey arrows indicate the vector field and red arrows are exemplary trajectories from initial conditions indicated by a grey dot. Corresponding time series plots for unstable subsystems 1 ( e ) and 2 ( f ), and the result of combining e and f to produce ( g ) system 3 (pathogen–predator–pest). The parameter values are: r =0.46, α 1 =0.9, α 2 =0.06, β 1 =1, β 2 =0.01, m 1 =0.47, m 2 =0.1, K =10 and ε =0.8, and the initial conditions are S 0 =1, I 0 =3 and L 0 =1 r is the per capita growth rate of the pest, α 1 and α 2 are the attack rates of the pathogen and the predator, respectively, β 1 and β 2 are the handling times of the pathogen and predator, respectively, m 1 and m 2 are the mortality rates of the pathogen and predator, respectively, K is the carrying capacity of the predator and ε is the conversion rate of infected prey consumed to predators produced. Full size image Destabilizing the control agents In the case of the pathogen, loss of control, instability, is characterized by boom-bust dynamics in the pest, where the booms and busts grow in magnitude with each passing cycle until reaching some large limit much beyond tolerance thresholds ( Fig. 1b,e ). In the case of the predator, instability is characterized by exponential growth of the pest once the predator reaches its carrying capacity K , a non-renewable resource that limits predator growth due to intraspecific competition, that is, space or nesting habitat ( Fig. 1d,f ) [46] . Both kinds of dynamics are classic representations of instability in theoretical ecology [5] , [44] , [47] . Fortunately, the dynamic simplicity of our model creates clear boundaries for stable and unstable dynamics (instability criteria indicated in Methods), and allows us to dictate when control is lost (unstable) by manipulation of a few key parameters. We find that to destabilize the pathogen, we can reduce the rate at which pathogens infect susceptible pests—the attack rate ( α 1 ), increase the natural mortality rate of the pathogen ( m 1 ) or increase the time required for an infection to kill the host pest—the handling time ( β 1 ) (Methods, equation (6)). To destabilize the predator, we can increase the rate at which the pests grow ( r ), decrease the amount of nesting habitat or space for the predator—the carrying capacity ( K ), decrease the rate at which predators attack pests ( α 2 ) or increase the time required for an individual predator to find, kill and consume one pest—the handling time ( β 2 ) (Methods, equation (9)). Note that in both cases, instability (and thus pest outbreak) occurs when the control agent is weakened. We then take these two weak, unstable control agents, and further weaken them by coupling the two systems through exploitative competition over a shared susceptible pest resource and IGP (predator consumes healthy pests, infected pests and the pathogens inside the infected pests) (Methods, equations (3a)–(3c), , ). We find that there indeed exist conditions where coupling two unstable control agents through negative interactions leads to stable coexistence of the two control agents and rescue of biological control ( Fig. 1e–g ). Healthy pest populations are markedly reduced when the control agents are combined and can remain at these low, stable equilibria for long timescales ( Fig. 1e–g ). Recall that to create instability the control agents were first weakened. Thus, it is reasonable to expect that the combination of two weak control agents could rescue control, corresponding to well-known notions of species complementarity [14] , [15] , [16] . However, what is especially interesting is that control is rescued in spite of strong negative interactions imposed by IGP and the inherent competition that occurs when multiple agents share a resource (Methods, equations (3a)–(3c), , ). It is important to note that previous theoretical work has already shown that weak, stable consumer–resource interactions can help dampen chaotic oscillations that result from strong consumer–resource interactions [11] , [12] . When formulated so that one or both control-agent–pest pairs are stable to begin with, our models reproduce this same result (see Supplementary Figs 1 and 2 ). However, here we take the issue one step further by showing that stability can be rescued even when each component system is unstable to begin with, and even when strong negative interactions are used to couple the unstable components ( Fig. 1e–g ). Stability hotspots We constrained parameter values to biologically realistic values for rates, such that control-agent attack rates, handling times and mortality rates were 0< α 1 , α 2 , β 1 , β 2 , m 1 , m 2 <1, then overlaid regions of parameter space where each of the independent subsystems were unstable based on the instability criteria calculated in Methods (equations (6) and (9); Fig. 2a–c ). We strategically sampled values within each zone, paired them and determined the stability of the resulting complex system ( Fig. 2d , see Methods). We found that parameter values on the edges of the instability regions for each independent control agent were most likely to be tipped into stable control when the two agents were combined; 9 out of 10 successful parameter combinations included at least one edge set ( P =0.021, n =10, exact binomial test) ( Fig. 2d ). Increased sampling specifically for edge values revealed 13 additional successful combinations ( Fig. 2d , see Methods). Rescue of stability was heavily dependent on parameter sets that included predators with low handling times; 13 out of 13 successful parameter combinations involved an edge where β 2 →0, ( P <0.001, n =13, exact binomial test) ( Fig. 2d ). Low handling times allow the predator to quickly consume both healthy and infected pests, reducing pathogen densities through competition and IGP, respectively. In this way, the predator is able to prevent the pathogen from ever becoming an epidemic and overexploiting the pests, effectively damping the unstable oscillations of the pathogen subsystem ( Fig. 1 ). 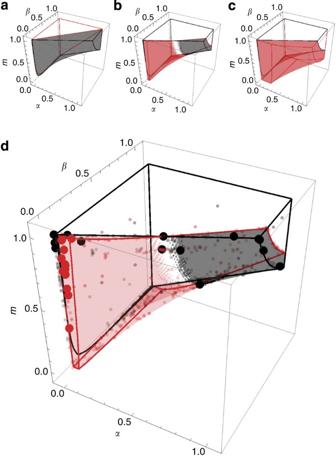Figure 2: Sampling of instability regions. Regions of three-dimensional parameter space that satisfy instability criteria for subsystem 1: pathogen–pest (black outline) (6), and subsystem 2: predator–pest (red outline) (9) overlaid. Control-agent attack rates (α), handling times (β) and mortality rates (m) are varied on each axis under conditions of (a) lowror highK(r=0.0001,K=10) or (r=0.46,K=6,000), (b) mediumrandK(r=0.46,K=10) and (c) highror lowK(r=0.99,K=4.5) or (r=0.46,K=2).ris the per capita growth rate of the pest, andKis the carrying capacity of the predator. Black-shaded region corresponds to parameter space where the pathogen is competitively dominant over the predator and the red-shaded region corresponds to parameter space where the predator is dominant over the pathogen based on parameter values ofα,βandm. (d) Strategically sampled unstable parameter sets for the pathogen (black dots) and predator subsystems (red dots) in the mediumrandKscenario. Larger dots represent unstable pathogen (black) and predator (red) parameter sets that successfully rescued stability in the combined, complex model (ε=0.8, conversion rate of infected pests into predator abundance). Figure 2: Sampling of instability regions. Regions of three-dimensional parameter space that satisfy instability criteria for subsystem 1: pathogen–pest (black outline) (6), and subsystem 2: predator–pest (red outline) (9) overlaid. Control-agent attack rates ( α ), handling times ( β ) and mortality rates ( m ) are varied on each axis under conditions of ( a ) low r or high K ( r =0.0001, K =10) or ( r =0.46, K =6,000), ( b ) medium r and K ( r =0.46, K =10) and ( c ) high r or low K ( r =0.99, K =4.5) or ( r =0.46, K =2). r is the per capita growth rate of the pest, and K is the carrying capacity of the predator. Black-shaded region corresponds to parameter space where the pathogen is competitively dominant over the predator and the red-shaded region corresponds to parameter space where the predator is dominant over the pathogen based on parameter values of α , β and m . ( d ) Strategically sampled unstable parameter sets for the pathogen (black dots) and predator subsystems (red dots) in the medium r and K scenario. Larger dots represent unstable pathogen (black) and predator (red) parameter sets that successfully rescued stability in the combined, complex model ( ε =0.8, conversion rate of infected pests into predator abundance). Full size image Relative strengths of agents By further adjusting the remaining parameters, pest growth rate ( r ) and predator carrying capacity ( K ), we note that there are only three general scenarios: the instability region of the predator is always underneath the instability region of the pathogen ( Fig. 2a ), the instability regions of each control agent overlap the other in some portion of phase space ( Fig. 2b ) and the instability region of the predator always overlaps the instability region of the pathogen ( Fig. 2c ). Considering that values on the edges of instability regions are more likely to rescue control, and larger instability regions extend towards higher attack rates, lower handling times and lower mortality rates (generally implying stronger control agents), the biological interpretation of these three scenarios are: the pathogen always beats the predator ( Fig. 2a ), equal competition ( Fig. 2b ) and the pathogen always loses to the predator ( Fig. 2c ). We know that rescue of stability is highly dependent on values near the edge of the predator instability region where β 2 →0 ( Fig. 2d ), and notice that this stability-inducing edge first appears when there is equal competition, and grows larger as the strength of the predator over the pathogen increases ( Fig. 2a–c ). The predator must effectively keep the pathogen from becoming an epidemic to rescue control, thus only the scenarios where there is equal competition between predator and pathogen or the predator always wins results in the rescue of biological control ( Fig. 2b,c ). We note that this can be achieved by increasing the growth rate of the pest ( r ) or decreasing the carrying capacity of the predator ( K ), which causes the instability region of the predator to increase in size, overlap the instability region of the pathogen and reveal the β 2 →0 edge that is so necessary in limiting the pathogen and rescuing control of the pest ( Fig. 2 ). Because the size of the β 2 →0 edge increases as the dominance of the predator over the pathogen increases, so too should the probability of successfully rescuing stability. Intraspecific versus interspecific competition One of the few general laws in ecology derived from the original Lotka–Volterra competition models suggests that intraspecific competition may need to be greater than interspecific competition if multiple enemies are to coexist in a biological control programme [8] . In our model, we implemented a carrying capacity in our predator to represent intraspecific competition over a non-renewable resource such as nesting habitat. The predator subsystem becomes unstable and loses control of the pest when nesting habitat is more limiting than pest resources, or when intraspecific competition is high. When the pathogen is introduced, strong competition over pests prevents the predator from reaching carrying capacity while also preventing the pathogen from overexploiting pests. This implies that interspecific competition becomes greater than intraspecific competition, yet coexistence is maintained. Although our model is based largely on the original Lotka–Volterra equations [44] , beginning with unstable components leads us to conclude that coexistence is maintained when interspecific competition is greater than intraspecific, the exact opposite of the classical outcome. Strength of IGP We note that our analysis here is not an exhaustive search of parameter space, but is intended to show the potential for stability to result spontaneously from the coupling of unstable components. By analysing each component system separately and keeping all parameters constant when combined, we can confidently assert that each system begins as a purely unstable unit, and that stability arises solely from the negative interactions that couple the independent units together. We refrain from adjusting parameters post combination, because doing so would alter the initial stability of the component systems. Our analysis is therefore constrained to parameters that are unique to the combined system, the only one being the conversion rate of infected pests into predator offspring ( ε ) (Methods, equations (3a)–(3c), , ). The cost of IGP (consumption of infected pests) to the predator is controlled by the parameter ε . Since the conversion rate of healthy pests into predator abundance is set to 1, an ε value <1 implies that the predator produces fewer offspring when consuming infected rather than healthy prey (Methods, equations (3a)–(3c), , ). We justify this by the fact that infected prey are less healthy by definition and arguably less nutritious, especially if predators are themselves susceptible to infection [7] , [26] . Time series data for varying ε show the existence of two major attractors, one where the peak abundances of predator and pathogen are synchronous ( Fig. 3a,b,d ) and one where they are asynchronous ( Fig. 3c,e ). The model is set up such that the predator consumes both uninfected/susceptible ( S ) and infected pests ( I ) with a constant attack rate ( α 2 ). At very low ε values, consumption of infected pests contributes little to predator recruitment, essentially acting like empty calories. Although the predator does not distinguish between healthy and infected pests directly, its population growth depends mainly on the number of healthy pests available, thus as the healthy pest population grows, so does the predator population. This results in synchrony between the predator and pathogen populations, since both depend primarily on healthy pests for recruitment. We call this the pathogen-dominant attractor, since the pathogen exerts a strong negative effect on the predator by reducing predator recruitment, and the dynamics mimic the cyclic instability of the pathogen-only subsystem ( Figs 1b and 4a ). As ε values approach 1, consumption of infected pests and healthy pests become equally important for predator recruitment. This causes the predator to synchronize with both healthy and infected pest populations, and a resulting asynchrony between predator and pathogen populations ( Fig. 4a ). We call this the predator-dominant attractor since there is almost no cost of IGP to the predator. By adjusting initial conditions and overlaying the resulting bifurcation plots, we can visualize the two interwoven attractors and see clear signs of hysteresis [48] , [49] , where position on one or the other attractor depends on the initial conditions of the system ( Fig. 5 ). A shift from one attractor to the other could result in a sudden increase in pest numbers resembling a regime shift, but this would only be considered a pest outbreak if pest tolerance thresholds were set particularly low (~11 for Fig. 5 ) [49] . It is important to note that for all of these simulations, the susceptible pest population remains bound to a very low range of possible values that are much below our original threshold of 500. This implies that the rescue of control from the combination of unstable agents is robust to perturbations in initial conditions and epsilon ( Fig. 5 ). In other words, stability is robust. 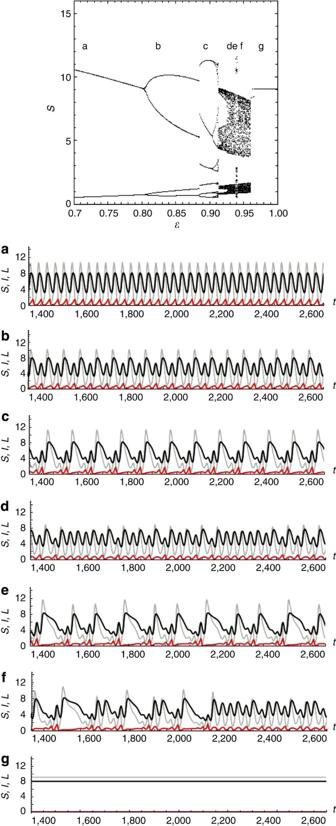Figure 3: Symmetric and asymmetric dynamical behaviour. Bifurcation diagram for conversion rate parameterεin system 3 varied from 0.70 to 1.00 evaluated for equilibrium values of the susceptible pest populationS, and corresponding time series graphs plotted for (a)ε=0.70, (b) 0.85, (c) 0.90, (d) 0.93, (e) 0.94, (f) 0.96 and (g) 1.00. Grey lines are number of susceptible pestsS, black lines are predatorsLand red lines represent infected pests or pathogensI. Ina,banddbehavior is symmetric (pathogen dominant), incandeasymmetric (predator dominant) andfmixed. All other parameter values are:r=0.46,α1=0.9,α2=0.06,β1=1,β2=0.01,m1=0.47,m2=0.1 andK=10, and the initial conditions areS0=1,I0=3 andL0=1.ris the per capita growth rate of the pest,α1andα2are the attack rates of the pathogen and the predator, respectively,β1andβ2are the handling times of the pathogen and predator, respectively,m1andm2are the mortality rates of the pathogen and predator, respectively andKis the carrying capacity of the predator. Figure 3: Symmetric and asymmetric dynamical behaviour. Bifurcation diagram for conversion rate parameter ε in system 3 varied from 0.70 to 1.00 evaluated for equilibrium values of the susceptible pest population S , and corresponding time series graphs plotted for ( a ) ε =0.70, ( b ) 0.85, ( c ) 0.90, ( d ) 0.93, ( e ) 0.94, ( f ) 0.96 and ( g ) 1.00. Grey lines are number of susceptible pests S , black lines are predators L and red lines represent infected pests or pathogens I . In a , b and d behavior is symmetric (pathogen dominant), in c and e asymmetric (predator dominant) and f mixed. All other parameter values are: r =0.46, α 1 =0.9, α 2 =0.06, β 1 =1, β 2 =0.01, m 1 =0.47, m 2 =0.1 and K =10, and the initial conditions are S 0 =1, I 0 =3 and L 0 =1. r is the per capita growth rate of the pest, α 1 and α 2 are the attack rates of the pathogen and the predator, respectively, β 1 and β 2 are the handling times of the pathogen and predator, respectively, m 1 and m 2 are the mortality rates of the pathogen and predator, respectively and K is the carrying capacity of the predator. 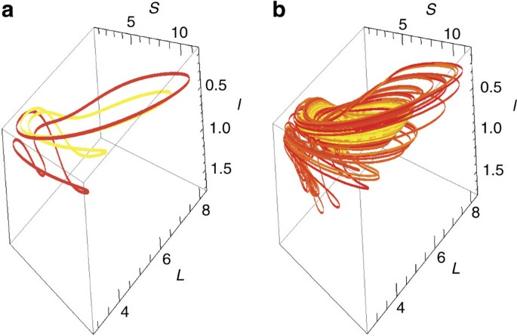Figure 4: Component and combined chaotic attractors. Pest abundance (S) plotted against pathogen (I)and predator abundance (L) yields three-dimensional phase portraits for system 3 ofa, two main attractors overlaid; symmetric, pathogen-dominant (yellow,ε=0.85), asymmetric, predator-dominant (red,ε=0.90), andb, chaotic attractor (ε=0.959) where colour is a function of position in phase space. All plots made using data fromt=5,000 to 10,000. Other parameter values are:r=0.46,α1=0.9,α2=0.06,β1=1,β2=0.01,m1=0.47,m2=0.1 andK=10, and the initial conditions areS0=1,I0=3 andL0=1.ris the per capita growth rate of the pest,α1andα2are the attack rates of the pathogen and the predator, respectively,β1andβ2are the handling times of the pathogen and predator, respectively,m1andm2are the mortality rates of the pathogen and predator, respectively,Kis the carrying capacity of the predator andεis the conversion rate of infected prey consumed to predators produced. Full size image Figure 4: Component and combined chaotic attractors. Pest abundance ( S ) plotted against pathogen ( I) and predator abundance ( L ) yields three-dimensional phase portraits for system 3 of a , two main attractors overlaid; symmetric, pathogen-dominant (yellow, ε =0.85), asymmetric, predator-dominant (red, ε =0.90), and b , chaotic attractor ( ε =0.959) where colour is a function of position in phase space. All plots made using data from t =5,000 to 10,000. Other parameter values are: r =0.46, α 1 =0.9, α 2 =0.06, β 1 =1, β 2 =0.01, m 1 =0.47, m 2 =0.1 and K =10, and the initial conditions are S 0 =1, I 0 =3 and L 0 =1. r is the per capita growth rate of the pest, α 1 and α 2 are the attack rates of the pathogen and the predator, respectively, β 1 and β 2 are the handling times of the pathogen and predator, respectively, m 1 and m 2 are the mortality rates of the pathogen and predator, respectively, K is the carrying capacity of the predator and ε is the conversion rate of infected prey consumed to predators produced. 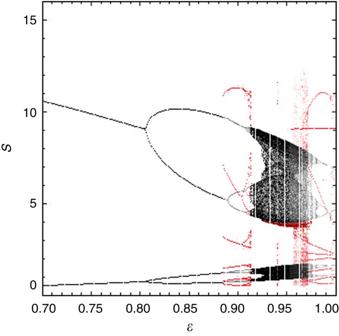Figure 5: Robust stability shown through bifurcation overlays. Conversion rate parameterεin system 3 is varied from 0.70 to 1.00 and evaluated for equilibrium values of the susceptible pest populationS.Overlay of 21 bifurcation diagrams plotted at 10% opacity, each initiated under different initial conditions and all other parameters kept constant. Putative predator-dominant attractor in red, pathogen-dominant attractor in black. Initial conditions ranged fromS0: 3 to 18,I0: 4 to 10 andL0: 11 to 13, chosen to reveal as much of each attractor as possible. The parameter values are:r=0.46,α1=0.9,α2=0.06,β1=1,β2=0.01,m1=0.47,m2=0.1 and andK=10.ris the per capita growth rate of the pest,α1andα2are the attack rates of the pathogen and the predator, respectively,β1andβ2are the handling times of the pathogen and predator, respectively,m1andm2are the mortality rates of the pathogen and predator, respectively,Kis the carrying capacity of the predator andεis the conversion rate of infected prey consumed to predators produced. Full size image Figure 5: Robust stability shown through bifurcation overlays. Conversion rate parameter ε in system 3 is varied from 0.70 to 1.00 and evaluated for equilibrium values of the susceptible pest population S. Overlay of 21 bifurcation diagrams plotted at 10% opacity, each initiated under different initial conditions and all other parameters kept constant. Putative predator-dominant attractor in red, pathogen-dominant attractor in black. Initial conditions ranged from S 0 : 3 to 18, I 0 : 4 to 10 and L 0 : 11 to 13, chosen to reveal as much of each attractor as possible. The parameter values are: r =0.46, α 1 =0.9, α 2 =0.06, β 1 =1, β 2 =0.01, m 1 =0.47, m 2 =0.1 and and K =10. r is the per capita growth rate of the pest, α 1 and α 2 are the attack rates of the pathogen and the predator, respectively, β 1 and β 2 are the handling times of the pathogen and predator, respectively, m 1 and m 2 are the mortality rates of the pathogen and predator, respectively, K is the carrying capacity of the predator and ε is the conversion rate of infected prey consumed to predators produced. Full size image At some values of ε in the predator–pathogen–pest system, trajectories may take the form of a complicated strange attractor, a bounded region from which all trajectories trace unique paths ( Fig. 4b ). Within the chaotic window, marked in the bifurcation plot as a dark band of infinitely many possible positions in phase space ( Fig. 5 ), we observe a strange attractor that switches between two modes reflecting the basic behaviour of the two attractors previously described ( Fig. 3f ). Thus, the strange attractor has three distinct phases: predator-dominant, pathogen-dominant and a phase that appears to be switching between the two ( Fig. 4 ). As each enemy appears to struggle to gain superiority over the shared resource, victory is always short-lived since both systems are unstable on their own. The winner always loses its advantage to the competitor, and the cycle repeats. Our formulation of system 3 assumes that the predator satiates at a rate dependent on the number of all prey available (type II functional response, typical for describing predators [50] ), with no discretion between infected or healthy prey (Methods, equations (3a)–(3c), , ). We note that altering the functional response of the predator so that it can distinguish infected and healthy prey simplifies the system such that the chaotic region shrinks, but the qualitative behaviour of rescuing stability remains the same ( Supplementary Fig. 3 ). We formulated the pathogen with a type III functional response [50] to be indicative of a pathogen within a spatially distributed population, where disease transmission is low when the host population is low and/or highly dispersed (since contact among individuals will be low) and transmission rapidly reaches some upper limit at high population densities once a critical density of hosts accumulates (Methods, equations (1a) and (1b)). Converting the functional response of the pathogen from type III to type II has similar consequences ( Supplementary Figs 4 and 5 ). It is also important to note that we can eliminate IGP and still rescue stability ( Supplementary Fig. 6 ), but the negative effects of competition over the shared resource can never be removed and thus are an inherent part of stabilizing system 3, making these results robust. When considering the efficiencies of two competing enemies simultaneously, we note that when the efficiency of one enemy is high the other must be low. In both the predator-dominant and pathogen-dominant attractors, the susceptible pest population peaks become more extreme as the negative effect of one enemy on the other increases. The paradox of biological control [5] (where attempts to increase efficiency of control may lead to the loss of biological control) occurs at both extremes, whether the predator (high ε ) or the pathogen (low ε ) is most efficient. The smallest oscillations occur at intermediate ε values in the chaotic region, when the efficiencies of the two competitors are more or less equal, and neither enemy has a competitive advantage over the other ( Fig. 5 ). If as is usually the case, the goal of management is to eliminate outbreaks, these results imply that strong, but fairly matched competition between enemies can help by minimizing pest population maximums. Thus, coupling two unstable systems with negative interactions has the counter-intuitive result of rescuing stability, creating a stable, more diverse system. Although usually suspected of hindering biological control and competitive coexistence, our results show potential for IGP and competition over shared resources to prevent outbreak dynamics and take unstable conditions to stable ones. In general, we found that strong interspecific competition can act as a stabilizing force if we begin with unstable components. These results can be tested empirically using laboratory populations of pests and control agents previously determined to be ineffective singularly. The overabundance of competitors and IGP in systems with effective autonomous biological control has always been difficult to explain, given the standard theory [1] , [2] , [3] , [4] , [5] , [6] , [7] , [27] , [28] . Here, we suggest that the prevalence of these negative interactions between diverse assemblages in nature may in fact contribute to the consistent and stable level of natural control found in many undisturbed ecosystems [3] , [27] , [28] , [30] , [51] . We add that evidence in favour of sampling effects from one strong natural enemy [16] , [17] , [18] , [19] , [20] are curiously also consistent with dominance hierarchies among competing enemies. An understanding of the stability of component parts apart from the system as a whole may be a necessary prerequisite to determining the consequence of strong negative interactions within complex networks. Model specifications Subsystem 1: pathogen–pest two-dimensional system based on the modified epidemic model [35] , where S is the number (not proportion) of susceptible pest individuals, I is the number of pest individuals infected by the pathogen and , a Holling type III functional response [50] . Subsystem 2: predator–pest two-dimensional system of equations based on the modified Rosenzweig/MacArthur model [34] altered to include density dependence on the predator [46] , where the predator is L (lady beetles), prey/pest is A (aphids), , a Holling type II functional response [50] and K is the carrying capacity of the predator, a non-renewable resource such as space or nesting habitat [46] . For these models, r is the per capita growth rate of the pest, α 1 and α 2 are the attack rates of the pathogen and the predator, respectively, β 1 and β 2 are the times necessary for the pathogen and predator, respectively, to search, kill, eat and otherwise handle one pest and m 1 and m 2 are the mortality rates of the pathogen and predator, respectively. System 3: combined pathogen–predator–pest three-dimensional system of equations, derived from A=S+I: The parameter ε is the conversion rate of infected pests into predator abundance. Since the conversion rate of healthy pests into predator abundance is effectively 1, when ε<1 , there is a reproductive cost to engaging in IGP for the predator. Stability analysis Subsystem 1: the pathogen (4a) and pest (4b) isoclines, where each respective population is at equilibrium or dI/dt =0 and dS/dt =0 are as follows: There exists one non-zero equilibrium point where the two isoclines overlap. The arrangement of the isoclines dictates whether this equilibrium point is stable or unstable, and in practical terms whether there is control or no control of the pest (equivalent to the classic ideas of epidemic or not). As the pathogen ( I) isocline becomes greater than the inflection point of the pest isocline (5, Fig. 1b ), the equilibrium point goes from exhibiting stable damped cycles to limit cycles of ever-increasing magnitudes. Rearranging (5) gives the following instability criteria for subsystem 1 (6), which can be achieved by reducing either the attack rate of the pathogen or increasing its mortality rate or handling time. Subsystem 2: the predator (7a) and pest (7b) isoclines, where dL/dt , dA/dt =0 are: There are two non-trivial equilibrium points where these isoclines overlap in positive space: one a stable point attractor exhibiting oscillatory behaviour and the other an unstable point repellor placed on a separatrix delimiting two basins of attraction (8) ( Fig. 1c ). A blue-sky bifurcation occurs when the slope or y -intercept of the pest isocline (7b) is increased such that the two equilibrium points collide ( Fig. 1d ), creating a half-stable point that eventually disappears ‘into the clear blue sky’ [47] . By setting the two equilibrium points equal to each other we can determine this exact point as the instability criteria for subsystem 2: Thus, increasing the growth rate of the pest r , lowering the carrying capacity of the predator K , increasing the handling time of the predator β 2 or decreasing the attack rate of the predator α 2 , can destabilize subsystem 2. All trajectories beyond this point are unstable as the predator reaches carrying capacity, and the pest continues to grow exponentially ( Fig. 1d ). Model testing Parameter sets for single control-agent components (subsystems 1 and 2) were strategically sampled within the instability regions calculated (equations (6) and (9)). Unstable parameter sets were then paired in the full model, system 3 (equations (3a)–(3c), , ), and resulting stability examined using time series data and bifurcation plots. All simulations where susceptible pest populations ( S ) were below a tolerance threshold of 500 individuals and neither predator, pathogen nor pest was eliminated after 10,000 time steps were considered stable. Strategic sampling To efficiently sample the unstable phase space of each control agent, 10 random parameter sets were pulled from (1) the entire instability region, (2) the edges bordering stability of the instability region (approaching the limits of the instability criteria—equations (6) and (9)) and (3) the region of the instability region that overlapped the instability region of the other control agent, which we will refer to as the dominant region. Predator parameter sets were fully crossed with pathogen sets, producing a total of 900 parameter combinations. Each of these parameter combinations was simulated for 10,000 time steps, and stability assessed for each. From the 10 successful combinations found, probability of rescuing stability based on region specificity was calculated using binomial exact tests. To refine which edges were important for rescuing stability, we separated the instability regions of each control agent into the six edges that border stability. These edges correspond to parameters approaching extreme values: α 1,2 →1, β 1,2 →1, β 1,2 →0, m 1,2 →1, m 1,2 →0, and the surface edge between unstable and stable regions where no particular parameter is at an extreme. Fifty additional parameter sets were randomly selected from each of the five extreme edges, and 100 from the surface edge for each control agent. The predator and pathogen parameter sets were then randomly matched, resulting in 350 total combinations. Each of these parameter sets was simulated, stability assessed and the probability of rescuing stability based on edge specificity calculated using binomial exact tests. Parameterization The parameter values for all plots are: r =0.46, α 1 =0.9, α 2 =0.06, β 1 =1, β 2 =0.01, m 1 =0.47, m 2 =0.1, K =10 and ε =0.8, and the initial conditions are S 0 =1, I 0 =3 and L 0 =1, unless otherwise noted. r is the per capita growth rate of the pest, α 1 and α 2 are the attack rates of the pathogen and the predator, respectively, β 1 and β 2 are the handling times of the pathogen and predator, respectively, m 1 and m 2 are the mortality rates of the pathogen and predator, respectively, K is the carrying capacity of the predator and ε is the conversion rate of infected prey consumed to predators produced. Bifurcation plots To examine the effects of variables of interest ( ε , f ) on system dynamics, models were run for 10,000 time steps, and population peaks estimated where the first derivative of the dynamical variable of interest (in most cases, S , the susceptible pest population) was naught. To remove transience, the last 20% of values were plotted for all bifurcations. How to cite this article : Ong, T. W. and Vandermeer, J. H. Coupling unstable agents in biological control. Nat. Commun. 6:5991 doi: 10.1038/ncomms6991 (2015).